Control of early seedling development by BES1/TPL/HDA19-mediated epigenetic regulation ofABI3 Seed germination and young seedling establishment should be tightly regulated to maximize plant survival and thereby enable successful propagation. Plants have evolved developmental signalling networks to integrate environmental cues for proper control of these critical processes, in which brassinosteroids are known to attenuate ABA-mediated arrest of early seedling development; however, the underlying regulatory mechanism remains elusive. Here we reveal that a BES1/TPL/HDA19 repressor complex mediates the inhibitory action of brassinosteroids on ABA responses during early seedling development. BR-activated BES1 forms a transcriptional repressor complex with TPL-HDA19, which directly facilitates the histone deacetylation of ABI3 chromatin. This event leads to the transcriptional repression of ABI3 and consequently ABI5 , major ABA signalling regulators in early seedling development. Our data reveal that the BR-activated BES1-TPL-HDA19 repressor complex controls epigenetic silencing of ABI3 and thereby suppresses the ABA signalling output during early seedling development. As sessile plants, the control of early seedling developmental processes, including seed germination and young seedling establishment, is central to the survival and successful propagation of the plant. Owing to high vulnerability to a vast array of stresses in early seedling developmental processes, multiple environmental and intrinsic signalling factors are intricately integrated to finely control these developmental processes. The signalling networks that integrate brassinosteroids (BRs), gibberellin (GA), abscisic acid (ABA) and light signals are important factors in the regulation of seed development, dormancy, germination and post-germinative developmental processes [1] , [2] , [3] , [4] . ABA plays important regulatory roles in maintaining seed dormancy and early seedling developmental arrest checkpoints [5] . ABI3 is an important regulatory factor for these ABA responses during early seedling development [6] , [7] , [8] , [9] . ABI3 loss-of-function mutations led to severe ABA insensitiveness in seed germination and abnormal embryonic development [8] , [10] , [11] . ABI3 directly enhanced the expression of ABI5 , encoding a major ABA signalling transcription factor, during early seedling development [12] . Interestingly, ABI3 mRNA contains a long 5′-untranslated region (UTR) and its partial truncation highly induced pABI3-GUS expression in seedlings [11] . Furthermore, ABI3 expression was highly increased in histone deacetylases HDA6/HDA19 RNA interference seedlings or by histone deacetylase inhibitor treatment [13] . These results indicate yet unknown negative regulation on the ABI3 promoter at the post-transcriptional level, probably by histone modification via HDA6 and 19. The key roles of GA and light signalling in attenuating the ABA responses during early seedling development have long been known [4] , and recent studies have revealed the essential functions of BR signalling pathways in the regulation of GA- and light-mediated plant development [1] , [3] . Exogenous BR application rescued the low germination phenotype of GA-related mutants and BR-defective mutants are hypersensitive to ABA during early seedling development and stomatal closure [14] , [15] , [16] . Furthermore, the biologically active BR (brassinolide and castasterone) and BR biosynthetic gene expression were greatly increased during seed growth and germination of Pisum sativum (pea) [17] . BR signalling cascades are initiated from the plasma membrane-anchored co-receptors BRI1 and BAK1 (refs 18 , 19 ). BR signalling dynamically regulates the activity of BR-related transcriptional factors, including BES1 and BZR1, by modulating the activity of BIN2 kinase and PP2A phosphatase [20] . Recent studies have revealed the crucial roles of BR in integrating numerous developmental signalling pathways [20] , [21] . BR was reported to have antagonist effects on ABA signalling based on the findings that the BR-defective det2 , bri1 and bin2-1 mutants are hypersensitive to ABA during early seedling development [14] , [22] . Furthermore, ABI2-mediated ABA signalling pathways were shown to negatively control primary BR signalling outputs by facilitating BIN2 activity [16] , suggesting that the coordination of BR and ABA signalling is accomplished by the BIN2-regulated transcriptional activity of BES1 or BZR1. However, the molecular mechanisms that integrate BR signalling pathways with ABA signalling in early seedling development are largely unknown. Here we demonstrate that BR-activated BES1 attenuates ABA sensitivities in early seedling development by recruiting the TPL-HDA19 co-repressor. The TPL-HDA19 complex enabled the nuclear-localized active BES1 to repress ABI3 , an important regulator in ABA responses during early seedling development, by facilitating histone deacetylation. Based on these observations, we propose that BR signalling cascades repress ABA responses via BES1-TPL-HDA19 co-repressor-mediated epigenetic silencing of ABI3 . BES1 specifically inhibits ABA responses BR-defective dwf4 , bri1 and bin2-1 mutants showed hypersensitivity to ABA, suggesting that the antagonistic roles of BR in ABA signalling pathways could be mediated by BIN2 kinase or its downstream components. As BIN2 inactivates the transcriptional activity of BES1 and BZR1, we initially analysed the ABA sensitivity of gsk triple knockout ( bin2 bil1 bil2 loss-of-function), bes1-D and bzr1-1D mutants [23] , [24] , [25] , all of which harboured constitutively activated BES1 or BZR1, in seed germination and root growth inhibition of young seedlings. Interestingly, the bes1-D and gsk triple mutants were less sensitive to ABA during seed germination compared with their wild-type controls, En-2 and Ws-2, respectively. However, the seed germination rate of bzr1-1D , a constitutively activated gain-of-function BZR1 allele, was lower than that of Col-0 in the presence of ABA ( Fig. 1a ). Furthermore, the growth of bes1-D roots was barely inhibited by exogenously applied ABA, while bzr1-1D and BR-insensitive bri1 mutants displayed more severe root growth inhibition than the wild-type on exogenous ABA application ( Fig. 1b ). We next tested the expression levels of representative ABA-responsive genes, including RD29A , RD29B and ABI1 , in bes1-D and bzr1-1D seedlings in the absence or presence of ABA. The expression of ABA-responsive genes was greatly reduced in the bes1-D seedlings, but not in the bzr1-1D mutant. 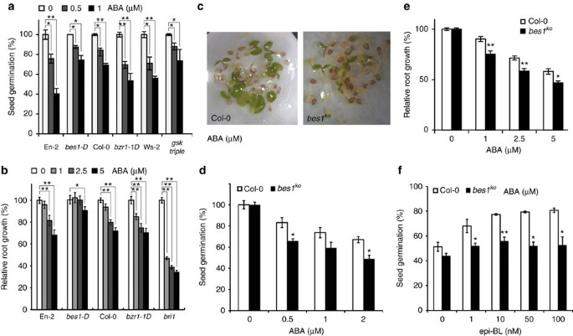Figure 1: BES1-mediated BR signalling specifically inhibits ABA responses. (a) BRs inhibit ABA signalling specifically through BES1 functions, but not BZR1.bes1-D bzr1-1D gsktriple mutant seeds were germinated on 1/2 B5 agar plates containing 0, 0.5 or 1 μM of ABA for 4 days and the germinated seeds (radicle emergence) were counted (error bars indicate s.e.;n=3; over 50 seeds were analysed in each independent experiment). Col-0, En-2 and Ws-2 were used as wild-type control. (b)bes1-Dwas less sensitive to ABA in terms of root growth inhibition. Four-day-old seedlings ofbes1-D,bzr1-1Dandbri1were transferred onto 1/2 B5 agar plate containing 0, 1, 2.5 or 5 μM ABA. Root length was measured after another 5 days, and relative growth was compared with that of seedlings grown on ABA-free medium (error bars indicate s.e.n>30). (c,d)bes1knockout (bes1ko) mutants are hypersensitive to ABA in seed germination. Seven-day-old seedlings ofbes1kogrown on 1/2 B5 medium containing 1 μM ABA (d).bes1koseeds were germinated on 1/2 B5 agar plates containing 0, 0.5 or 1 μM ABA for 3 days and the germinated seeds (radicle emergence) were counted (d); error bars indicate s.e.;n=3; over 50 seeds were tested in each independent experiment). (e) ABA-mediated inhibition of root growth was increased inbes1ko. Four-day-old seedlings ofbes1koand Col-0 were transferred onto 1/2 B5 agar plates containing 0, 1, 2.5 or 5 μM ABA. Root length was measured after another 5 days and growth was compared with that on ABA-free medium (error bars indicate s.e.;n>30). (f) The inhibitory effects of BRs on ABA responses during seed germination were rarely observed in thebes1komutant. Seed germination rates of the wild type andbes1kogrown on 1 μM of ABA with 0, 1, 10, 50 and 100 nM epi-BL 4 days after plating (error bars indicate s.e.;n=3; over 100 seeds were tested in each independent experiment). Asterisks indicate statistically significant differences analysed by Student’st-test (*P<0.05, **P<0.01). However, both bes1-D- and bzr1 -1D- expressing plants exhibited lower expression levels of the BR biosynthetic genes, CPD and DWF4 ( Supplementary Table 1 ). Moreover, ABA-induced activation of the ABA-responsive genes was greatly reduced in the bes1-D seedlings ( Supplementary Table 1 ). In bzr1-1D seedlings, however, RD29A and ABI1 were expressed at similar levels as in wild-type plants, and exogenously applied ABA greatly enhanced the accumulation of RD29B ( Supplementary Table 1 ). Furthermore, exogenously applied BR completely suppressed the hypersensitive ABA response of bzr1-1D -expressing plants in germination, similar to the wild-type control ( Supplementary Fig. 1a ). These results suggest that BR-mediated suppression of ABA signalling is specifically controlled by BES1, but not by BZR1, in spite of their similar roles in BR signalling pathways. Figure 1: BES1-mediated BR signalling specifically inhibits ABA responses. ( a ) BRs inhibit ABA signalling specifically through BES1 functions, but not BZR1. bes1-D bzr1-1D gsk triple mutant seeds were germinated on 1/2 B5 agar plates containing 0, 0.5 or 1 μM of ABA for 4 days and the germinated seeds (radicle emergence) were counted (error bars indicate s.e. ; n =3; over 50 seeds were analysed in each independent experiment). Col-0, En-2 and Ws-2 were used as wild-type control. ( b ) bes1-D was less sensitive to ABA in terms of root growth inhibition. Four-day-old seedlings of bes1-D , bzr1-1D and bri1 were transferred onto 1/2 B5 agar plate containing 0, 1, 2.5 or 5 μM ABA. Root length was measured after another 5 days, and relative growth was compared with that of seedlings grown on ABA-free medium (error bars indicate s.e. n >30). ( c , d ) bes1 knockout ( bes1 ko ) mutants are hypersensitive to ABA in seed germination. Seven-day-old seedlings of bes1 ko grown on 1/2 B5 medium containing 1 μM ABA ( d ). bes1 ko seeds were germinated on 1/2 B5 agar plates containing 0, 0.5 or 1 μM ABA for 3 days and the germinated seeds (radicle emergence) were counted ( d ); error bars indicate s.e. ; n =3; over 50 seeds were tested in each independent experiment). ( e ) ABA-mediated inhibition of root growth was increased in bes1 ko . Four-day-old seedlings of bes1 ko and Col-0 were transferred onto 1/2 B5 agar plates containing 0, 1, 2.5 or 5 μM ABA. Root length was measured after another 5 days and growth was compared with that on ABA-free medium (error bars indicate s.e. ; n >30). ( f ) The inhibitory effects of BRs on ABA responses during seed germination were rarely observed in the bes1 ko mutant. Seed germination rates of the wild type and bes1 ko grown on 1 μM of ABA with 0, 1, 10, 50 and 100 nM epi-BL 4 days after plating (error bars indicate s.e. ; n =3; over 100 seeds were tested in each independent experiment). Asterisks indicate statistically significant differences analysed by Student’s t- test (* P <0.05, ** P <0.01). Full size image Next, we determined the ABA sensitivity of the bes1 knockout ( bes1 ko ) mutant. Although the gain-of-function bes1-D plants had a lower sensitivity to ABA, the root growth and seed germination of the bes1 ko mutant displayed enhanced responses to ABA relative to wild-type plants ( Fig. 1c–e ), supporting the negative roles of BES1 in ABA signalling pathways. To verify that BES1 is required for BR-mediated suppression of ABA signalling outputs, we determined the effect of BR treatment on the germination of bes1 ko in the presence of ABA. Interestingly, although the ABA-mediated inhibition of seed germination in wild-type Col-0 was gradually abolished by exogenous BR (epi-BL) treatment in a dose-dependent manner, the effects of ABA on seed germination in bes1 ko were barely affected by exogenous BR ( Fig. 1f ). Furthermore, exogenous BR application gradually suppressed ABA-mediated inhibition of early seedling development of wild-type in a BR dosage-dependent manner, but bes1 ko seedlings were barely responded to exogenous BR for early development in the presence of ABA ( Supplementary Fig. 1b ). Taken together, we conclude that BES1-mediated BR signalling pathways specifically attenuate ABA signalling during early seedling development. BR-activated BES1 represses ABI3 expression Our results showed that BR signalling pathways attenuated ABA responses through the activity of BES1, and the expression of representative ABA-responsive genes was greatly reduced in bes1-D seedlings, suggesting that BES1 negatively regulates the expression of ABA signalling-related genes. Recent studies also reported that BES1 represses the expression of several target genes [26] , [27] , [28] . To test this idea, we determined the expression levels of ABA signalling-related genes in a gain-of-function bes1-D and bes1 ko plants using real-time quantitative reverse transcription–PCR (qRT–PCR). Interestingly, the expression of major transcription factors of the ABA signalling pathway, including ABF s, ABI3 and ABI5 , was greatly decreased in bes1-D seedlings ( Fig. 2a ); however, ABF1 , ABI3 and ABI5 were upregulated in bes1 ko seedlings ( Fig. 2b ). Notably, ABI3 and ABI5 , central ABA signalling components in the regulation of early seedling development, were upregulated in bes1 ko seedlings ( Fig. 2b ). As the expression of ABI5 is enhanced by ABI3 (ref. 12 ), we propose that BR-activated BES1 regulates the ABI3-ABI5-mediated ABA signalling module. Consistently, exogenously applied BR decreased the concentration of ABI3 transcripts in wild-type seedling in a time- and dose-dependent manner, but the expression of ABI3 barely changed in bes1 ko in response to BR ( Fig. 2c ). These results suggest that BES1 has an important role in the BR-mediated repression of ABI3 . 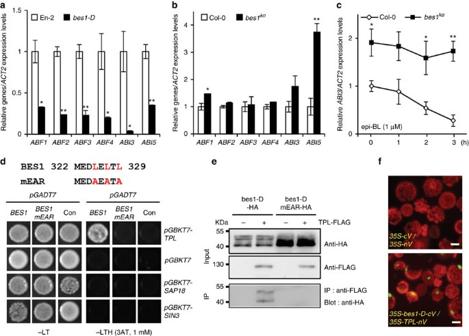Figure 2: BES1-TPL repressor complexes are involved in the BR-mediated repression ofABI3. (a,b) The expression of ABA-related transcription factors is regulated by BES1. The expression levels ofABF1-4,ABI3,ABI4andABI5in 4-day-oldbes1-D(a) andbes1koseedlings (b) were determined by real time qRT–PCR (error bars indicate s.e.;n=4). (c) BR treatment downregulatesABI3expression. The expression levels ofABI3in 4-day-old Col-0 andbes1koseedlings treated with 1 μM epi-BL for 1, 2 and 3 h were determined by real-time qRT–PCR (error bars indicate s.e.;n=4). (d) BES1 interacts with TPL via its EAR motif, but not with SIN3 or SAP18. Core residues of the EAR motif sequence of BES1 are indicated in red (L×L×L) and the sequence is aligned with that of mutated EAR (three core Leu substitute to Ala, mEAR; upper). Yeast cells transformed with the indicated gene sets were selected in synthetic medium lacking Leu, Trp (-LT) or His (-LTH), but containing 1 mM 3AT. (e) bes1-D-HA proteins co-immunoprecipitated with FLAG-tagged TPL. Mesophyll protoplasts were transfected withbes1-D-HAandbes1-DmEAR-HAwithTPL-FLAG, incubated for 6 h and then pulled down with anti-FLAG antibodies. bes1-D proteins were detected with anti-HA antibody. (f) TPL interacts with BES1 in the nucleus. BiFC (bimolecular fluorescence complementation) assay using TPL-nV (nVenus) and cV (cVenus)-tagged bes1-D. Scale bar, 50 μM. Asterisks indicate statistically significant differences analysed by Student’st-test (*P<0.05, **P<0.01). Figure 2: BES1-TPL repressor complexes are involved in the BR-mediated repression of ABI3 . ( a , b ) The expression of ABA-related transcription factors is regulated by BES1. The expression levels of ABF1-4 , ABI3 , ABI4 and ABI5 in 4-day-old bes1-D ( a ) and bes1 ko seedlings ( b ) were determined by real time qRT–PCR (error bars indicate s.e. ; n =4). ( c ) BR treatment downregulates ABI3 expression. The expression levels of ABI3 in 4-day-old Col-0 and bes1 ko seedlings treated with 1 μM epi-BL for 1, 2 and 3 h were determined by real-time qRT–PCR (error bars indicate s.e. ; n =4). ( d ) BES1 interacts with TPL via its EAR motif, but not with SIN3 or SAP18. Core residues of the EAR motif sequence of BES1 are indicated in red ( L × L × L ) and the sequence is aligned with that of mutated EAR (three core Leu substitute to Ala, mEAR; upper). Yeast cells transformed with the indicated gene sets were selected in synthetic medium lacking Leu, Trp (-LT) or His (-LTH), but containing 1 mM 3AT. ( e ) bes1-D-HA proteins co-immunoprecipitated with FLAG-tagged TPL. Mesophyll protoplasts were transfected with bes1-D-HA and bes1-DmEAR-HA with TPL-FLAG , incubated for 6 h and then pulled down with anti-FLAG antibodies. bes1-D proteins were detected with anti-HA antibody. ( f ) TPL interacts with BES1 in the nucleus. BiFC (bimolecular fluorescence complementation) assay using TPL-nV (nVenus) and cV (cVenus)-tagged bes1-D. Scale bar, 50 μM. Asterisks indicate statistically significant differences analysed by Student’s t- test (* P <0.05, ** P <0.01). Full size image We next investigated how BR-activated BES1 repressed ABI3 . Recently, EAR (ethylene-responsive element binding factor-associated amphiphilic repression) motif-mediated transcriptional repression mechanisms have been reported, and many transcriptional repressors use this mechanism to regulate plant developmental programmes [29] , [30] . In the primary structure of BES1, we identified a putative EAR motif (LxLxL) ( Fig. 2d ) essential for recruiting Groucho/Tup1-like transcriptional co-repressors, such as TPL, SAP18 and SIN3 (refs 31 , 32 ). To verify that BES1 interacts with transcriptional co-repressors via the EAR motif, we performed a yeast two-hybrid assay with BES1 and its EAR mutant (mEAR; Fig. 2d , upper). Interestingly, TPL interacted with bes1-D and BES1, as well as a positive control IAA3 (ref. 30 ), but mutations of the EAR motif of BES1 or a dominant negative tpl-1 (N176H) mutation disrupted these protein interactions in yeast ( Fig. 2d and Supplementary Fig. 2a,b ). However, SAP18 and SIN3 were not associated with bes1-D or BES1 ( Fig. 2d and Supplementary Fig. 2a ). The Arabidopsis genome has four TPL-RELATED genes ( TPR1–4 ). We found that TPR2 could also interact with BES1 but not TPR3, and the amino-terminal domain of TPL, TPR1, TPR2 and TPR4 was enough to bind with BES1 ( Supplementary Fig. 2c,d ). These imply that TPL and its closely related TPRs might have functional redundancy in the formation of the co-repressor complex with BES1. We next investigated the protein interactions between TPL and BES1 by in vivo co-immunoprecipitation assays. The wild-type BES1 proteins are highly phosphorylated and mostly localized at cytosols in plants [33] , but TPL proteins are mainly localized in the nucleus [30] . Furthermore, both phosphorylated and dephosphorylated BES1 proteins interacted with TPL-N ( Supplementary Fig. 3a ). Therefore, for the in vivo interaction assay, we used the constitutively activated bes1-D proteins, which are mostly dephosphorylated and located in the nucleus. Whereas bes1-D-HA proteins were pulled down by TPL-FLAG, bes1-DmEAR proteins were not ( Fig. 2e ). We also found that bes1-D and TPL interacted in the nucleus ( Fig. 2f ). Finally, BR enhanced the interaction of BES1 with TPL in the nucleus ( Supplementary Fig. 3b ). These results indicate that BES1-TPL/TPR1/2/4 could form a transcriptional co-repressor complex that plays important roles in BES1-mediated ABI3 repression. BES1–TPL complex regulates both BR and ABA responses To further explore whether the BES1-TPL complex is involved in the BR-mediated suppression of ABA responses, we generated 35S-bes1-DmEAR-HA lines and examined ABA-related seed germination and root growth inhibition ( Fig. 3a,b and Supplementary Fig. 4 ). We selected four independent lines in which bes1-DmEAR-HA proteins were highly accumulated ( Supplementary Fig. 4a ). Interestingly, the 35S-bes1-DmEAR-HA lines did not show any BR-related phenotypes, including curled rosette leaves and brassinazole resistance in hypocotyl elongation, which were generally displayed in bes1-D- overexpressing plants ( Supplementary Fig. 4b,c ). However, the BR-related phenotypes were completely recovered in bes1-DmEAR by its protein fusion with SRDX (the EAR repression domain), TPL or TPL-binding HDA19 at the carboxy terminus ( Supplementary Fig. 5a,b ). These results indicate that the formation of repressor complex with TPL/HDA19 is essential for the BES1-mediated regulation of BR-related plant growth and development. We next investigated the ABA responses in 35S-BES1-HA , 35S-bes1-DmEAR , 35S-bes1-DmEAR-TPL and 35S-bes1-DmEAR-HDA19 lines. Interestingly, although 35S-bes1-D was less sensitive to ABA in terms of seed germination and root growth inhibition than wild-type or 35S-BES1-HA plants, mutation of the EAR motif of bes1-D disrupted ABA tolerance ( Fig. 3a,b and Supplementary Fig. 4d ). Consistent with activated BR responses, the 35S-bes1-DmEAR-TPL and 35S-bes1-DmEAR-HDA19 lines showed less sensitivity to ABA in root growth inhibition, similar to bes1-D mutant, than Col-0 ( Supplementary Fig. 5c ). Consistently, the expression of ABI3 , ABI5 and AtEm6 was reduced in bes1-DmEAR-HDA19 -overexpressing plants but upregulated in the bes1-D-mEAR -overexpressing lines compared with wild-type plants. Moreover, BR biosynthesis-related CPD and DWF4 were also significantly reduced in bes1-D- and bes1-DmEAR-HDA19 -overexpressing plants ( Supplementary Fig. 5d ). Taken together, we conclude that BES1 represses ABI3 expression through the EAR-mediated recruitment of the TPL-HDA19 co-repressor. 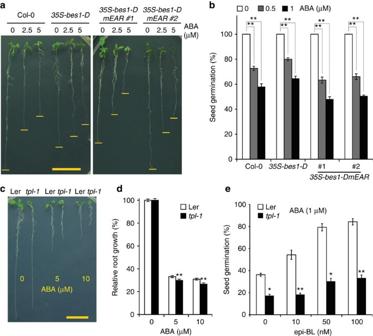Figure 3: BES1-TPL co-repressors function in the BR-mediated inhibition of ABA signalling. (a,b) The EAR motif of BES1 is required for repressing ABA responses. Four-day-old seedlings of Col-0,35S-bes1-Dand35S-bes1-DmEAR(lines 1 and 2) were transferred onto 1/2 B5 agar plates containing 0, 2.5 or 5 μM ABA. Scale bar, 10 mm. (a) Col-0,35S-bes1-Dand35S-bes1-DmEAR(1 and 2) mutant seeds were germinated on 1/2 B5 agar plates containing 0, 0.5 or 1 μM ABA for 4 days and the germinated seeds (radicle emergence) were counted (b); error bars indicate s.e.;n=3; over 50 seeds were tested in each independent experiment). (c,d) A dominant negativetpl-1mutant was hypersensitive to ABA in terms of root growth inhibition. Four-day-old seedlings oftpl-1and the wild type (Ler) were transferred onto 1/2 B5 agar plates containing 0, 5 or 10 μM ABA. Scale bar, 10 mm. (c) Root length was measured after another 5 days and growth was compared with that on ABA-free medium (d), error bars indicate s.e.;n>60). (e) Germination of thetpl-1mutant scarcely responds to BRs in the presence of ABA. Seed germination rates of the wild type andtpl-1mutants grown on 1 μM ABA with 0, 10, 50 and 100 nM epi-BL 4 days after plating (error bars indicate s.e.;n=3; over 100 seeds were tested in each independent experiment). Asterisks indicate statistically significant differences analysed by Student’st-test (*P<0.05, **P<0.01). Figure 3: BES1-TPL co-repressors function in the BR-mediated inhibition of ABA signalling. ( a , b ) The EAR motif of BES1 is required for repressing ABA responses. Four-day-old seedlings of Col-0, 35S-bes1-D and 35S-bes1-DmEAR (lines 1 and 2) were transferred onto 1/2 B5 agar plates containing 0, 2.5 or 5 μM ABA. Scale bar, 10 mm. ( a ) Col-0, 35S-bes1-D and 35S-bes1-DmEAR (1 and 2) mutant seeds were germinated on 1/2 B5 agar plates containing 0, 0.5 or 1 μM ABA for 4 days and the germinated seeds (radicle emergence) were counted ( b ); error bars indicate s.e. ; n =3; over 50 seeds were tested in each independent experiment). ( c , d ) A dominant negative tpl-1 mutant was hypersensitive to ABA in terms of root growth inhibition. Four-day-old seedlings of tpl-1 and the wild type (Ler) were transferred onto 1/2 B5 agar plates containing 0, 5 or 10 μM ABA. Scale bar, 10 mm. ( c ) Root length was measured after another 5 days and growth was compared with that on ABA-free medium ( d ), error bars indicate s.e. ; n >60). ( e ) Germination of the tpl-1 mutant scarcely responds to BRs in the presence of ABA. Seed germination rates of the wild type and tpl-1 mutants grown on 1 μM ABA with 0, 10, 50 and 100 nM epi-BL 4 days after plating (error bars indicate s.e. ; n =3; over 100 seeds were tested in each independent experiment). Asterisks indicate statistically significant differences analysed by Student’s t- test (* P <0.05, ** P <0.01). Full size image To decipher the functions of the BES1-TPL complex in the BR-mediated suppression of ABA signalling outputs, we tested the ABA responses during early seedling development in a semi-dominant negative tpl-1 mutant. As expected, compared with wild-type plants, the root elongation of tpl-1 seedlings was significantly reduced by exogenously applied ABA (5 and 10 μM; Fig. 3c,d ). Moreover, the germination rate of tpl-1 was significantly lower than in the wild type in the presence of 1 μM ABA ( Fig. 3e ), suggesting that TPL functions are negatively associated in ABA signalling pathways. To examine whether TPL functions were connected with the BR-mediated suppression of ABA signalling, we determined the effect of BR application on the germination of tpl-1 in the presence of ABA. In the presence of 1 μM ABA, the inhibitory effect of ABA on the germination of wild-type seeds was rescued by exogenously applied BR in a dose-dependent manner. However, the BR-mediated inhibition of the effects of ABA on seed germination was barely observed in tpl-1 ( Fig. 3e ). Consistently, ABI3 and ABI5 transcripts were highly accumulated in tpl-1 seedlings compared with wild-type ( Supplementary Fig. 6 ). Together, these results suggest that TPL-mediated repression of its target genes is involved in the coordination of BR and ABA signalling pathways in early seedling development. BES1-TPL-HDA19 co-repressors directly target ABI3 chromatin To elucidate whether the BES1-TPL complex could directly repress ABI3 , we carried out a chromatin immunoprecipitation (ChIP) assay using a pBES1-bes1-D-HA transgenic line. We found several BES1-binding E-box sequences (CAnnTG) [28] in a ~3-kb upstream region of the ABI3 promoter containing the 5′-UTR region ( Fig. 4a , upper green ovals and Supplementary Fig. 7 ). The bes1-D-HA proteins strongly bound to BES1-binding elements (E-box) on the 5′-UTR (6) and a promoter region (1) of the ABI3 locus, as well as the SAUR-AC1 promoter region used as a positive control ( Fig. 4a ). However, we did not observe any differences in the DNA binding of bes1-D and bzr1-1D to the other tested promoter regions (2–5; Fig. 4a ). We further confirmed the BES1 binding to 1 and 6 regions of the ABI3 promoter by electrophoretic mobility shift assays ( Supplementary Fig. 8 ). These results indicate that BES1 could directly repress ABI3 transcription by binding to the 5′-UTR and a promoter region. In agreement with these results, it was previously reported that the 5′-UTR region of ABI3 is essential for the negative regulation of its transcription [11] . However, we could not find the direct binding of BES1 to the ABI5 promoter ( Supplementary Fig. 9 ). We next tested whether the BES1-binding E-box motifs in the ABI3 promoter is required for BR-mediated repression of ABI3 . A mutation of E-box motifs on either 1 or 6 regions could not block the bes1-D-mediated repression of pABI3-LUC activity [4] , but double mutations of the E-box motifs on both 1 and 6 regions ( pABI3m-LUC ) abolished the repression of the ABI3 promoter activity by bes1-D ( Supplementary Fig. 10a ). We then generated GUS -expressing transgenic plants under the control of either wild-type ABI3 ( pABI3-GUS ) or mutated ABI3 promoter ( pABI3m-GUS ). Exogenous ABA induced GUS expression of both pABI3-GUS and pABI3m-GUS lines ( Supplementary Fig. 10b ). Interestingly, however, exogenous BR repressed GUS expression of the pABI3-GUS transgenic lines, but not of the pABI3m-GUS lines ( Fig. 4b and Supplementary Fig. 10c,d ). Conversely, the expression of endogenous CPD and ABI3 was reduced by BR treatment in both pABI3-GUS and pABI3m-GUS lines ( Supplementary Fig. 10c,d ). To further investigate whether BES1-mediated repression of ABI3 is functionally important for BR action on ABA signalling, we generated pABI3-gABI3-FLAG and pABI3m-gABI3-FLAG transgenic lines in the ABA-insensitive abi3-8 mutant background [34] . We selected two independent abi3-8 pABI3-gABI3-FLAG and pABI3m-gABI3-FLAG transgenic lines in which the ABA insensitiveness of abi3-8 in seed germination was fully restored to wild-type level ( Supplementary Fig. 11a ). However, ABA inhibition of seed germination in the abi3-8 pABI3m-gABI3-FLAG lines was barely suppressed by exogenous BR, but in abi3-8 pABI3-gABI3-FLAG lines and wild-type control ( Fig. 4c and Supplementary Fig. 11b ). These results indicate that BR specifically targets ABI3 expression via BES1, which is critical for determining ABA responsiveness during early seedling development. 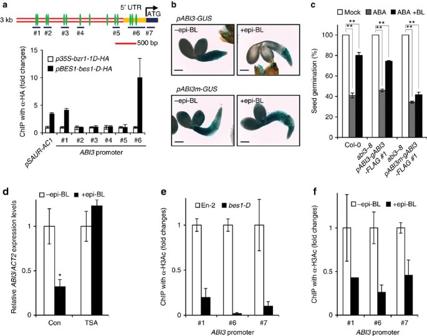Figure 4: BR decreases histone H3 acetylation on theABI3locus via BES1-TPL-HDA19 co-repressor complexes. (a) BES1 directly binds to the 5′-UTR and promoter ofABI3. ChIP assays of theABI3promoter and 5′-UTR were performed with anti-HA antibody. Schematic structure of theABI3promoter (3 kb). Putative E-Boxes (CAnnTG) and the 5′-UTR are marked with green ovals and yellow box, respectively (upper panel). The fold enrichments are presented as relative levels to an internal control,35S-bzr1-1D-HA(error bars indicate s.e.;n=3). TheSAUR-AC1promoter was used as a positive control. (b) BR treatment repressesGUSexpression driven by wild-typeABI3promoter, but not by mutatedABI3promoter. Three-day-old seedlings ofpABI3-GUS(upper) andpABI3m-GUS(lower) lines incubated with (+epi-BL) or without 1 μM BR (-epi-BL) for 3 h were stained with GUS solution. Scale bar, 200 μM. (c) BR barely suppress ABA responsiveness ofabi3-8 pABI3m-gABI3-FLAGlines in seed germination, but that ofabi3-8 pABI3-gABI3-FLAGlines. Seed germination (radicle emergence) rates were determined in the wild-type (Col-0),abi3-8 pABI3-gABI3-FLAGandabi3-8 pABI3m-gABI3-FLAGline grown on 0 (Mock) or 1 μM ABA with 0 (ABA) or 100 nM epi-BL (ABA+BL) for 3 days after plating (error bars indicate s.e.;n=3; over 100 seeds were tested in each independent experiment). (d) Trichostatin A (TSA) inhibits the BR-mediated repression ofABI3. The expression levels ofABI3in 4-day-old seedlings treated with 1 μM epi-BL for 3 h after pretreatment of 5 μM TSA for 24 h were determined by real-time qRT–PCR (error bars indicate s.e.;n=4). (e) ChIP analysis of the acetylation states of histone H3 in theABI3locus of wild-type andbes1-Dplants. ChIP assays using an anti-acetyl-histone H3 antibody were performed, and the fold enrichments were normalized with the En-2 control (error bars indicate s.e.;n=3). (f) BR treatment decreases the acetylation of histone H3 in theABI3locus. ChIP assays using an anti-acetyl-histone H3 antibody were performed on 4-day-old wild-type seedlings treated with or without 1 μM epi-BL for 3 h, and the fold enrichments were normalized with mock treatment control (error bars indicate s.e.;n=3). Asterisks indicate statistically significant differences analysed by Student'st-test (*P<0.05, **P<0.01). Figure 4: BR decreases histone H3 acetylation on the ABI3 locus via BES1-TPL-HDA19 co-repressor complexes. ( a ) BES1 directly binds to the 5′-UTR and promoter of ABI3 . ChIP assays of the ABI3 promoter and 5′-UTR were performed with anti-HA antibody. Schematic structure of the ABI3 promoter (3 kb). Putative E-Boxes (CAnnTG) and the 5′-UTR are marked with green ovals and yellow box, respectively (upper panel). The fold enrichments are presented as relative levels to an internal control, 35S-bzr1-1D-HA (error bars indicate s.e. ; n =3). The SAUR-AC1 promoter was used as a positive control. ( b ) BR treatment represses GUS expression driven by wild-type ABI3 promoter, but not by mutated ABI3 promoter. Three-day-old seedlings of pABI3-GUS (upper) and pABI3m-GUS (lower) lines incubated with (+epi-BL) or without 1 μM BR (-epi-BL) for 3 h were stained with GUS solution. Scale bar, 200 μM. ( c ) BR barely suppress ABA responsiveness of abi3-8 pABI3m-gABI3-FLAG lines in seed germination, but that of abi3-8 pABI3-gABI3-FLAG lines. Seed germination (radicle emergence) rates were determined in the wild-type (Col-0), abi3-8 pABI3-gABI3-FLAG and abi3-8 pABI3m-gABI3-FLAG line grown on 0 (Mock) or 1 μM ABA with 0 (ABA) or 100 nM epi-BL (ABA+BL) for 3 days after plating (error bars indicate s.e. ; n =3; over 100 seeds were tested in each independent experiment). ( d ) Trichostatin A (TSA) inhibits the BR-mediated repression of ABI3 . The expression levels of ABI3 in 4-day-old seedlings treated with 1 μM epi-BL for 3 h after pretreatment of 5 μM TSA for 24 h were determined by real-time qRT–PCR (error bars indicate s.e. ; n =4). ( e ) ChIP analysis of the acetylation states of histone H3 in the ABI3 locus of wild-type and bes1-D plants. ChIP assays using an anti-acetyl-histone H3 antibody were performed, and the fold enrichments were normalized with the En-2 control (error bars indicate s.e. ; n =3). ( f ) BR treatment decreases the acetylation of histone H3 in the ABI3 locus. ChIP assays using an anti-acetyl-histone H3 antibody were performed on 4-day-old wild-type seedlings treated with or without 1 μM epi-BL for 3 h, and the fold enrichments were normalized with mock treatment control (error bars indicate s.e. ; n =3). Asterisks indicate statistically significant differences analysed by Student's t -test (* P <0.05, ** P <0.01). Full size image Several prior studies suggested that RPD3-like histone deacetylase 19 (HDA19) was directly recruited to TPL to actively repress gene expression [35] , [36] . To test whether the activity of HDA19 is responsible for the BES-mediated ABI3 repression, we determined the effects of Trichostatin A, a histone deacetylase-specific inhibitor, on BR-induced ABI3 repression. As shown in Fig. 4d , BR treatment significantly reduced ABI3 expression, but this effect was completely abolished by Trichostatin A treatment. HAD19 activity is an important regulator of histone H3 and H4 acetylation in plants [35] , [37] , indicating that BR could decrease histone acetylation states on the ABI3 chromatin via the BES1-recruited TPL-HDA19 co-repressor complex. To test this idea, we performed a ChIP assay using an anti-acetyl-Histone H3 antibody in bes1-D and BR-treated wild-type and bes1 ko seedlings. The histone H3 acetylation states in the BES1-binding regions of the ABI3 promoter (1 and 6) and the first exon region (7) were greatly reduced in the bes1-D and BR-treated wild-type seedlings compared with controls ( Fig. 4e,f ). However, BR-mediated reduction in histone H3 acetylation states of the ABI3 promoter was mostly impaired in bes1 ko seedlings ( Supplementary Fig. 11c ). Together, these results imply that BR directly induces the epigenetic silencing of ABI3 via the BES1-TPL complex. BR signalling is directly linked to the ABI3-ABI5 module To confirm the BES1-mediated epigenetic silencing of ABI3 in plants, we overexpressed HA (haemagglutinin)-tagged ABI3 or its downstream target, ABI5 , in the bes1-D background and determined the ABA responses in seed germination and root growth inhibition. We first tested the expression levels of ABI3-HA and ABI5-HA proteins in the bes1-D transgenic lines using an anti-HA antibody ( Fig. 5a and Supplementary Fig. 12a ). We selected four and two independent ABI3-HA (3–6) and ABI5-HA (12 and 18) overexpressing lines, respectively, among several T3 homozygous plants. As expected, the overexpression of ABI3 or ABI5 completely abolished the reduced ABA sensitivity phenotype of bes1-D plants in seed germination and root growth inhibition ( Fig. 5b–d and Supplementary Fig. 12b ). Especially, the ABA sensitivity of ABI3-HA -overexpressing bes1-D lines in seed germination was highly correlated with the ABI3-HA expression levels ( Fig. 5b ). Moreover, in the root growth inhibition assay, the bes1-D 35S-ABI3-HA transgenic seedlings (lines 5 and 6) were hyper-responsive to ABA treatment, while the ABA response was greatly reduced in bes1-D plants ( Fig. 5b–d ). However, the weak ABI3-HA-expressing plants (lines 3 and 4) revealed milder ABA sensitivity than the wild type, but their responses to ABA in the root growth inhibition assay were more sensitive than those of bes1-D seedlings ( Fig. 5d ). These results fully support the idea that BES1-mediated ABA repression occurs through the suppression of ABI3/ABI5 -mediated ABA signalling modules. 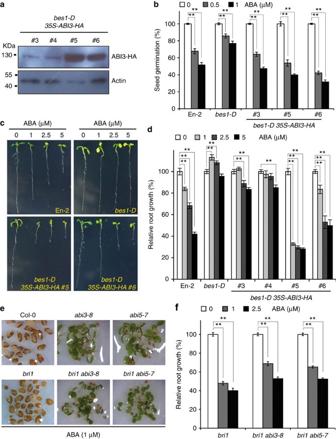Figure 5: BES1-mediated BR signalling is integrated into the ABI3-ABI5 module of ABA signalling. (a) ABI3 levels inABI3-HA-overexpressingbes1-Dlines (3–6). The protein expression levels of ABI3-HA inbes1-D 35S-ABI3-HAlines were detected with an anti-HA antibody. Actin was used as a loading control. (b) Ectopic expression of ABI3 eliminates the reduced sensitivity ofbes1-1Dto ABA. En-2,bes1-Dand three independentbes1-D 35S-ABI3-HAtransgenic seeds (3, 4 and 6) were germinated on the 1/2 B5 agar plates containing 0, 0.5 or 1 μM ABA for 4 days and the germinated seeds (radicle emergence) were counted (error bars indicate s.e.;n=3; over 50 seeds were tested in each independent experiment). (c,d) Ectopic expression of ABI3 suppresses the ABA-insensitive root phenotype ofbes1-1D. Four-day-old35S-ABI3-HA(3–6),bes1-Dand En-2 seedlings were transferred to 1/2 B5 agar plate containing 0, 1, 2.5 or 5 μM ABA. Representative35S-ABI3-HAtransgenic (5 and 6),bes1-Dand En-2 seedlings grown on the ABA containing media for 5 days. (c) Five days later, root length was measured and relative growth was compared with that of plants grown on ABA-free medium (d), error bars indicate s.e.;n>30). (e) The ABA hypersensitivity ofbri1in seed germination was completely suppressed by theabi3-8orabi5-7mutation. Five-day-oldbri1 abi3-8andbri1 abi5-7double mutant seedlings grown on 1/2 B5 medium containing 1 μM ABA. (f) ABA-mediated root growth inhibition assay usingbri1 abi3-8andbri1 abi5-7seedlings. Four-day-old Col-0,bri1,bri1 abi3-8andbri1 abi5-7seedlings were transferred onto 1/2 B5 agar plates containing 0, 1 or 2.5 μM ABA. Root length was measured after a further 5 days and relative growth was compared with that of plants grown on ABA-free medium (error bars indicate s.e.;n>30). Asterisks indicate statistically significant differences analysed by Student’st-test (**P<0.01). Figure 5: BES1-mediated BR signalling is integrated into the ABI3-ABI5 module of ABA signalling. ( a ) ABI3 levels in ABI3-HA -overexpressing bes1-D lines (3–6). The protein expression levels of ABI3-HA in bes1-D 35S-ABI3-HA lines were detected with an anti-HA antibody. Actin was used as a loading control. ( b ) Ectopic expression of ABI3 eliminates the reduced sensitivity of bes1-1D to ABA. En-2, bes1-D and three independent bes1-D 35S-ABI3-HA transgenic seeds (3, 4 and 6) were germinated on the 1/2 B5 agar plates containing 0, 0.5 or 1 μM ABA for 4 days and the germinated seeds (radicle emergence) were counted (error bars indicate s.e. ; n =3; over 50 seeds were tested in each independent experiment). ( c , d ) Ectopic expression of ABI3 suppresses the ABA-insensitive root phenotype of bes1-1D . Four-day-old 35S-ABI3-HA (3–6), bes1-D and En-2 seedlings were transferred to 1/2 B5 agar plate containing 0, 1, 2.5 or 5 μM ABA. Representative 35S-ABI3-HA transgenic (5 and 6), bes1-D and En-2 seedlings grown on the ABA containing media for 5 days. ( c ) Five days later, root length was measured and relative growth was compared with that of plants grown on ABA-free medium ( d ), error bars indicate s.e. ; n >30). ( e ) The ABA hypersensitivity of bri1 in seed germination was completely suppressed by the abi3-8 or abi5-7 mutation. Five-day-old bri1 abi3-8 and bri1 abi5-7 double mutant seedlings grown on 1/2 B5 medium containing 1 μM ABA. ( f ) ABA-mediated root growth inhibition assay using bri1 abi3-8 and bri1 abi5-7 seedlings. Four-day-old Col-0, bri1 , bri1 abi3-8 and bri1 abi5-7 seedlings were transferred onto 1/2 B5 agar plates containing 0, 1 or 2.5 μM ABA. Root length was measured after a further 5 days and relative growth was compared with that of plants grown on ABA-free medium (error bars indicate s.e. ; n >30). Asterisks indicate statistically significant differences analysed by Student’s t- test (** P <0.01). Full size image BR signalling-defective mutants displayed enhanced responses to ABA in seed germination and root growth inhibition of young seedlings ( Fig. 1 ). To determine if BRI1-triggered BR signalling pathways genetically interact with ABI3/ABI5-mediated ABA signalling modules, we crossed the bri1 knockout mutant to the loss-of-function abi3-8 and abi5-7 . Interestingly, the enhanced ABA sensitivity of bri1 in seed germination was completely suppressed by abi3-8 and abi5-7 mutations ( Fig. 5e and Supplementary Fig. 12c ). Furthermore, the abi3-8 or abi5-7 mutation significantly reduced the enhanced ABA responses of bri1 in root growth inhibition ( Fig. 5f and Supplementary Fig. 12d ). Finally, we found that DWF4- overexpressing seeds ( dwf4-D ) were also resistant to a GA biosynthetic inhibitor, paclobutrazol, during germination ( Supplementary Fig. 13 ). These results support that the ABA signalling module via ABI3 and ABI5 is directly regulated by BR signalling pathways. Taken together, we propose that BR-activated BES1 signalling pathway reduces the expression of ABI3 and consequently its downstream target, ABI5 , a key ABA signalling component that inhibits seed germination and young seedling growth ( Supplementary Fig. 14 ). The regulation of plant seed germination and young seedling establishment has both ecological and economic importance [4] . Diverse environmental factors, including light quality, water availability and temperature, are co-ordinately integrated into hormonal regulatory pathways that control early seedling development. Light signals induce the transition from heterotrophic to autotrophic growth of young seedlings by inhibiting skotomorphogenesis. In particular, BR is an essential factor for promoting the skotomorphogenic developmental programmes of germinated seedlings [20] . Furthermore, BR has recently been shown to have important roles in light-, GA- and temperature-mediated regulation of plant development [38] , [39] , suggesting the crucial biological relevance of BR in coordinating diverse signalling cues during early seedling development. In this study, we demonstrate the key roles of BES1-mediated BR signalling pathways in modulating the ABA responses during early seedling development. As germinated embryos and young seedlings are so vulnerable to variable environmental conditions, germination and stress tolerance of seedlings are expected to be regulated by elaborate mechanisms. The stress hormone ABA has long been considered as a major factor in the regulation of seed dormancy and stress tolerance. Indeed, under unfavourable conditions, such as desiccation and high salinity, ABA activity is greatly elevated in young seedlings, which maximizes stress tolerance, but arrests the seed-to-young seedling transition [5] . This growth checkpoint is known to be affected by the transcription factor ABI5, which is accumulated in response to ABI3, ABI4 and DWA1/2 (refs 40 , 41 ), which confer not only osmo-tolerance to the germinated young seedlings, but also upregulate a number of critical genes that arrest the growth of the germinated seedlings [12] . The expression of ABI5 is upregulated by ABI3, and ABI3 itself can also directly regulate the expression of key negative regulators involved in the seed-to-seedling transition [42] . These results indicate that the ABI3-ABI5 signalling module acts as a central negative regulator of early seedling development, and that factors that promote the seed-to-seedling transition should attenuate ABI3/ABI5-mediated ABA signalling module. Consistently, the drastic downregulation of ABI3 and ABI5 was observed on seed imbibition and the loss-of-function mutation of ABI3 and ABI5 disrupted ABA-mediated young seedling growth arrest [5] , [12] . Our work provides compelling evidence for the crucial roles of BES1 in the BR-mediated suppression of ABA responses via direct repression of the ABI3-ABI5 signalling module in early seedling development. BR-activated BES1 directly binds to the ABI3 promoter, but not to the ABI5 promoter, and represses its expression by reducing histone acetylation at ABI3 chromatin by recruiting TPL-HDA19 co-repressor complexes ( Figs 2 , 3 , 4 ). BRs promote cell elongation and inhibit photomorphogenesis, and these physiological features are also commonly regulated by GA. There are multiple overlaps in the gene sets regulated by BR and GA, and in the biological effects of these two hormones, and the BR-regulated transcriptional activity of BZR1 and BES1 is known to be required for proper GA responses in skotomorphogenic seedlings [1] , [3] . In addition, similar to GAs, BRs play negative roles in ABA-inhibited early seedling development [14] , [15] , [16] , and exogenous BR application or overexpression of BR biosynthetic DWF4 can overcome the low seed germination phenotype of GA-defective mutants [43] . Furthermore, central negative regulators of GA signalling, DELLA proteins, could directly inhibit the transcriptional activity of BES1 and BZR1, and BR activity was required for GA-mediated cell elongation [1] , [3] . Collectively, these results suggest that GA signalling is integrated with the BES1-mediated repression of ABI3 , to stimulate early seedling development. In addition, exogenous BR application dramatically increased tolerance to diverse abiotic stresses [44] , [45] , indicating that the increased BR activity during early seedling development could promote seedling hardiness without arresting growth. BES1 and BZR1 repress several target genes, including BR biosynthetic genes, light signalling components and chloroplast development-related genes [46] , [47] . However, it has been an open question as to how these two transcription factors repress their target genes. Epigenetic reprogramming of gene expression through DNA methylation, histone modification and chromatin remodelling without the alteration of nucleotides provides a flexible means of regulating gene expression and coordinating developmental programmes in eukaryotic organisms [48] . Plant-specific EAR motif-mediated epigenetic transcriptional repression has recently emerged as a key mechanism for modulating numerous hormonal, stress and developmental signalling pathways [29] . In this study, we show that the repressor activity of BES1, which is mediated by TPL-HDA19 co-repressor complexes, is essential for BR-mediated plant growth and development ( Figs 2 and 3 and Supplementary Figs 2–5 ). Interestingly, the EAR motif is evolutionarily conserved in all BR-related transcription factors, including BZR1 and BEH1-4 of Arabidopsis and other plant species. This suggests that TPL-mediated epigenetic histone remodelling mechanisms have critical roles in BR-mediated gene regulation and plant development. Histone methylation is frequently followed by deacetylation, which condenses chromatin into a structure that is highly repressive to gene transcription [49] . Interestingly, TPL could also interact with histone methylation-related chromatin remodellers, including SUVH3 (SUV39H-like protein) and PKR1 (PICKLE homologue) [29] . Thus, the BR-related transcription factors can also use diverse chromatin remodelling mechanisms to repress their target genes. However, BES1, together with its binding partner, can also act as a transcriptional activator [28] , [50] . BES1 can directly increase the demethylation of several target chromatins, including TCH4 , by recruiting two Jumonji family histone demethylases, ELF6 (Early flowering 6) and REF6 (Relative of early flowering 6). The elf6 and ref6 loss-of-function mutations resulted in a semi-dwarf phenotype and enhanced the growth defects of bri1-5 (ref. 50 ). Moreover, recent studies showed that BR and ELF6 affected flowering time [51] , [52] , indicating that by recruiting ELF6 and REF6, and functioning as a transcriptional activator, BES1 coordinates flowering and BR signalling pathways. BR signalling pathways have important roles in plant morphogenesis and many signalling stimuli are integrated into BR-mediated plant development [20] . Therefore, the context-dependent switching of BES1 and its homologues between transcriptional activators and repressors plays fundamental roles in the BR-dependent coordination of multiple signalling networks. The ubiquitous expression of BES1 (ref. 25 ) suggests that the switching of BES1 properties is achieved by the tissue-specific expression or post-transcriptional/translational modification of its binding factors, such as TPL, ELF6 and REF6. The context-dependent regulation of gene expression in multicellular organisms imparts biological diversity and specificity to transcription factors, which may aid in accomplishing developmental programmes. It will be very interesting to determine how these multiple chromatin remodelling mechanisms facilitate BR-mediated plant growth and development. Plant materials and growth conditions Arabidopsis thaliana ecotype Col-0, En-2, Ler and WS-2 were used as wild-type controls and as the genetic backgrounds of transgenic lines. Arabidopsis seeds were germinated in media (pH 5.7) containing 1/2 × Gamborg B5 salts (Duchefa, Haarlem, The Netherlands), 1% sucrose and 0.8% phytoagar under long-day conditions (16-h light/8-h dark cycles) at 22–24 °C. The mutant seeds were kindly provided by Dr Sunghwa Choe at the Seoul National University ( bes1-D , bzr1-1D , dwf4-D and bri1 ), Dr Jianming Li at the University of Michigan ( gsk triple), Dr Zhi-Yong Wang at the Carnegie Institution for Science ( bes1 knockout) and Dr Eiji Nambara at University of Toronto ( abi3-8 and abi5-7 ). tpl-1 seeds (CS65909) were provided by The Arabidopsis Biological Research Center. To generate bri1 abi3-8 (L298F) or bri1 abi5-7 (W75 Stop) mutants, genetic crosses were performed and double mutants were confirmed by DNA sequencing with gene-specific primer sets ( Supplementary Table 2 ). Protein–protein interaction assay To identify interactions between BES1 and co-repressors (TPL, TPR2, TPR3, SIN3 or SAP18), AH109 yeast strains were co-transformed with pGBKT7- co-repressors ( TPL , tpl-1 , TPR2 , TPR3 , SIN3 or SAP18 ) and pGADT7-BES1 ( bes1-D ). For interaction test of BES1 with N-terminal domain of TPL, TPR1, TPR2 or TPR4, 600 bp of the coding region of each gene was cloned into the pGBKT7 vector. Clones showing positive interactions were selected on synthetic medium containing 1 mM 3-aminotriazole without Leu, Trp and His. For the bimolecular fluorescence complementation and co-immunoprecipitation assays, TPL , BES1 or bes1-D-mEAR was cloned into a plant expression vector containing nV (nVenus, 1–157 amino acids), cV (cVenus, 158–238 amino acids), HA, myc or FLAG tags in the C terminus driven by the 35S C4PPDK promoter as previously described [53] , [54] . The Venu s gene (NCBI accession number BAJ39289) for bimolecular fluorescence complementation assay was provided by Professor Inhwan Hwang at POSTECH. For protoplasts transient expression assays in protoplasts, 4 × 10 4 protoplasts were transfected with 20–40 μg of plasmid DNA purified by CsCl-gradient ultracentrifugation and then incubated under constant light at 23 °C for 6 h. For BR treatment, the transfected protoplasts with BES1-cV and TPL-nV were further incubated for 3 h in the presence of 1 μM of epi-BL. The complemented Venus fluorescence was observed using a fluorescence microscope (Axioplan, Carl Zeiss MicroImaging, Inc.). For co-immunoprecipitation, total protein was extracted from the transfected protoplasts in IP buffer (50 mM Tris, pH 7.5, 75 mM NaCl, 5 mM EDTA, 1% Triton X-100, protease inhibitor cocktail (Roche), 1 mM dithiothreitol) and incubated with 1/100 dilutions of a monoclonal anti-myc (Cell Signaling, catalogue number 2276) or FLAG (Sigma, catalogue number F1804) antibody. The protein–antibody complex was precipitated with Protein A/G PLUS-Agarose beads (Calbiochem). Immunoprecipitated proteins were subjected to SDS–PAGE (10% polyacrylamide) and blotted onto polyvinylidene difluoride membranes (Millipore). The blots were probed with 1/2,000 dilution of a peroxidase-conjugated anti-HA antibody (Roche,catalogue number 12013819001), anti-FLAG antibody (Sigma, catalogue number A8592) or a monoclonal anti-myc antibody. All experiments were repeated three times with similar results. Transgenic plants and immunoblotting assay To generate transgenic plants overexpressing HA-tagged ABI3 and ABI5 in the bes1-D background, genomic DNAs were cloned into pCB302ES containing the 35S promoter and HA tag sequences as described previously [53] , [54] . For bes1-DmEAR -overexpressing plants, bes1-DmEAR was subcloned into pCB302ES . For pABI3-GUS and pABI3-gABI3-FLAG lines, 3-kb of the ABI3 promoter was cloned into either pCAMBIA1303 containing β-glucronidase ( GUS ) or pBI121 containing two copies of FLAG epitope-tagged genomic ABI3 . Four putative BES1-binding E-box motifs (CAnnTG) located at −278~284, −321~327, −336~342 and −2,496~2,502 in the ABI3 promoter were mutated to AAnnTG generating pABI3m-GUS and pABI3m-gABI3-FLAG lines. All transgenes were integrated into the Arabidopsis genome by Agrobacterium -mediated floral dipping. The transgene expression was verified by immunoblotting with 1/2,000 dilution of a monoclonal anti-HA antibody (Roche, catalogue number 12013819001). Total proteins from protoplasts or seedlings were extracted with protein extraction buffer (50 mM Tris-HCl (pH 7.5), 75 mM NaCl, 5 mM EDTA, 1 mM dithiothreitol, 1 × protease inhibitor cocktail (Roche) and 1% Triton X-100). Next, 3–20 μg of proteins were separated by SDS–PAGE (10% polyacrylamide), transferred to a polyvinylidene difluoride membrane and immunodetected using 1/2,000 dilution of peroxidase-conjugated high-affinity anti-HA (Roche), peroxidase-conjugated anti-FLAG (Sigma, catalogue number A8592) and anti-actin (MP Biomedicals, catalogue number 69100) antibodies. Full scans of all western blottings are provided in Supplementary Fig. 15 . Real-time qRT–PCR analysis To determine the expression levels of transcripts, total RNA was isolated from 3- to 4-day-old seedlings using Trizol reagent (Invitrogen). Double-strand complementary DNA was synthesized from 1 μg RNA with oligo dT primers and ImProm-II reverse transcriptase (Promega). Quantitative real-time PCR was performed with 1 μl of cDNA and gene-specific primer sets according to the instructions provided for the Light Cycler 2.0 (Roche) and the SYBR Taq Premix system (Takara/Enzynomics) with the following condition: total 45 cycles of denaturation at 95 °C for 15 s, annealing at 57 °C for 20s and extension at 72 °C for 13~25 s. ACT2 was used as an internal control. The data analysis and fold-change calculation was done with the delta Ct method [55] , [56] provided for the Light Cycler 2.0 software. The sequences of all gene-specific primers used in this study are listed in Supplementary Table 2 . Physiological analysis and histochemical GUS staining For seed germination assays, surface-sterilized homozygous seeds were kept at 4 °C for 4 days and plated on 1/2 Gamborg B5 medium containing 1% sucrose supplemented with or without the indicated concentrations of ABA or epi-BL. After 3 days, the seed germination (radicle emergence) rates were scored and normalized with those of the wild-type controls. For root elongation assays, 4-day-old seedlings grown vertically on Gamborg B5 medium containing 1% sucrose and 0.8% agar (pH 5.7) were transferred onto fresh medium (1.2% agar) containing various concentrations of ABA. The seedlings were further incubated for 5 days and the primary root lengths were measured. To investigate GUS expression patterns by BR treatments, 3-day-old seedlings of pABI3-GUS and pABI3m-GUS were incubated with 1 μM epi-BL (Sigma) for 4 h. The seedlings were stained with GUS-staining buffer (100 mM Tris-HCl (pH 7.0), 2 mM ferricyanide and 2 mM X-Gluc (5-bromo-4-chloro-3-indolyl-β- D -glucuronidase)) for 12 h. Chromatin immunoprecipitation ChIP assay was performed as previously described [57] . Five-day-old seedlings (~0.2 g) were harvested and immersed in cross-linking buffer (0.4 M sucrose, 10 mM Tris-HCl, pH 8.0, 1 mM EDTA, 1 mM phenylmethanesulphonylfluoride, 1% formaldehyde) under a vacuum for 10 min. Glycine was added to a final concentration of 0.1 M to stop the cross-linking and incubation was continued for 5 min under vacuum. The seedlings were ground in liquid nitrogen and resuspended in 1 ml of lysis buffer (50 mM HEPES, pH 7.5, 150 mM NaCl, 1 mM EDTA, 1% Triton X-100, 0.1% deoxycholate, 0.1% SDS, 1 × protease inhibitor cocktail (Roche)). DNA was sheared by sonication to ~500–1,000-bp fragments. After centrifugation, the supernatant was precleared with 40 μl salmon sperm DNA/Protein A/G agarose for 1 h at 4 °C. After centrifugation, the supernatant was diluted tenfold with dilution buffer (20 mM Tris-HCl, pH 8.0, 150 mM NaCl, 0.2 mM EDTA, 0.1% Triton X-100, 1 × protease inhibitor cocktail (Roche)) and transferred to 1.5 ml tubes. Next, 5 μl of the appropriate antibody (anti-HA (Roche, catalogue number 11867423001) or anti-acetyl-Histone H3 (Millipore, catalogue number 06-599)) was added, and the samples were incubated overnight at 4 °C. Next, 40 μl salmon sperm DNA/Protein A/G agarose was added to the samples and they were further incubated for 2 h at 4 °C. The beads were successively washed with 1 ml of 2 × lysis buffer, 2 × LNDET (0.25 M LiCl, 1% NP40, 1% deoxycholate, 1 mM EDTA, 10 mM Tris-HCl, pH 8.0) and 3 × TE (10 mM Tris-HCl, pH 8.0, 1 mM EDTA). The immunoprecipitated DNAs were eluted by adding 100 μl 10% Chelex 100 slurry, and analysed by quantitative real-time PCR. The sequences of primers used throughout this work are available in Supplementary Table 2 . How to cite this article: Ryu, H. et al. Control of early seedling development by BES1/TPL/HDA19-mediated epigenetic regulation of ABI3 . Nat. Commun. 5:4138 doi: 10.1038/ncomms5138 (2014).